The cell cycle regulator 14-3-3σ opposes and reverses cancer metabolic reprogramming Extensive reprogramming of cellular energy metabolism is a hallmark of cancer. Despite its importance, the molecular mechanism controlling this tumour metabolic shift remains not fully understood. Here we show that 14-3-3σ regulates cancer metabolic reprogramming and protects cells from tumorigenic transformation. 14-3-3σ opposes tumour-promoting metabolic programmes by enhancing c-Myc poly-ubiquitination and subsequent degradation. 14-3-3σ demonstrates the suppressive impact on cancer glycolysis, glutaminolysis, mitochondrial biogenesis and other major metabolic processes of tumours. Importantly, 14-3-3σ expression levels predict overall and recurrence-free survival rates, tumour glucose uptake and metabolic gene expression in breast cancer patients. Thus, these results highlight that 14-3-3σ is an important regulator of tumour metabolism, and loss of 14-3-3σ expression is critical for cancer metabolic reprogramming. We anticipate that pharmacologically elevating the function of 14-3-3σ in tumours could be a promising direction for targeted anticancer metabolism therapy development in future. Tumorigenesis is characterized by 10 hallmarks described by Hanahan and Weinberg [1] in their seminal paper. Among these, deregulation of cellular energetics (also called metabolic reprogramming) involves tumour cells ‘rewiring’ their metabolic pathways to support rapid proliferation, continuous growth, metastasis, survival and resistance to therapies [1] , [2] , [3] , [4] . Increases in glycolysis, glutaminolysis, lipid metabolism, mitochondrial biogenesis and energy production are among the most prominent metabolic alterations in cancer [1] , [2] , [3] , [5] , [6] , [7] , [8] , [9] . In fact, these processes provide tumours with not only energy but also essential precursors to support their biosynthesis and proliferation [2] , [5] , [10] . Cancer metabolism is regulated mainly by c-Myc (Myc), HIF1α, and p53 (refs 2 , 3 , 5 , 9 , 11 , 12 ). The interplay between these master regulators determines the status of tumour metabolism and has a decisive impact on tumorigenesis [2] . However, the regulation of cancer bioenergetics is not fully understood, suggesting that more regulators remain to be identified [3] , [13] . c-Myc (Myc) is frequently overexpressed in many human cancers. Myc is a major oncogenic transcription factor that can induce tumorigenesis by promoting cell proliferation, causing genome instability and blocking cell differentiation [14] . More importantly, Myc can also upregulate glycolytic genes, thereby promoting glucose consumption and glycolysis [2] , [15] . The upregulation of these glycolytic enzymes is due to Myc’s binding to its target genes for transcriptional activation [2] , [12] , [16] , [17] . In addition to glycolysis, Myc is the primary inducer of glutaminolysis in cells [11] , [17] , [18] . The metabolic switch to aerobic glycolysis and glutaminolysis is crucial to support Myc-mediated proliferation, growth, survival and metastasis of tumour cells. Despite the significant roles of Myc in many signalling pathways and cellular processes, the mechanism behind Myc regulation is not fully understood. 14-3-3 is an evolutionarily conserved family consisting of seven isoforms regulating many important cellular processes [19] . 14-3-3σ is the only one of the isoforms possessing tumour-suppressing ability, which is due to its unique structure [19] , [20] , [21] , [22] , [23] . 14-3-3σ is a direct target of p53 and protects p53 from MDM2-mediated ubiquitination and degradation [24] , [25] . 14-3-3σ is also a potent cell cycle regulator that inhibits the activity of Cdk2/cyclin E to cause arrest at the G 1 phase of the cell cycle and sequesters Cdc2/cyclin B to the cytoplasm to induce G 2 arrest [19] , [24] , [26] , [27] . The expression of 14-3-3σ is frequently lost in tumours of epithelial origin, including most breast cancers [19] , [21] . 14-3-3σ is silenced either by hypermethylation of the promoter of the Sfn gene, which encodes the 14-3-3σ protein [21] , or by increase in ubiquitin-mediated degradation of 14-3-3σ (refs 28 , 29 ). It is possible that 14-3-3σ loss leads to deregulations characterized in cancer hallmarks, including metabolic reprogramming. In this study, we show that the frequent loss of 14-3-3σ in cancer leads to the metabolic reprogramming phenotype that aids cancer growth and correlates with poor cancer survival. We demonstrate that 14-3-3σ mitigates tumour-promoting metabolic programmes by promoting c-Myc polyubiquitination and subsequent degradation, thereby reversing Myc-mediated cancer glycolysis, glutaminolysis and mitochondrial biogenesis in cancer. Our study discovers 14-3-3σ as an important regulator of cancer cellular energetics and holds the potential to unlock a door to new cancer treatment therapies. Loss of 14-3-3σ in cancer results in metabolic reprogramming Immunohistochemical analysis of breast tumour tissue microarrays and retrospective comparison with patient clinical data revealed that a low level of 14-3-3σ protein expression in breast tumours was significantly associated with poor survival ( Fig. 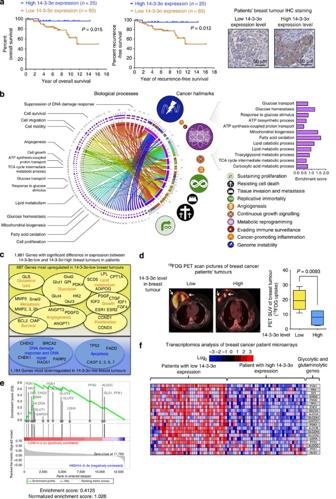Figure 1: The clinical relevance of 14-3-3σ in breast cancer and tumour metabolic reprogramming. (a) High 14-3-3σ expression was associated with prolonged breast cancer patients’ survival. 14-3-3σ protein expression levels in breast cancer patients at MD Anderson Cancer Center were evaluated using immunohistochemistry staining and matched with clinical data. 14-3-3σ protein expression in normal breast tissues was used as a reference to stratify patients. Log-rank test. (b) Downregulation of 14-3-3σ is associated with upregulation of major cancer hallmarks especially deregulation of cellular energetics (that is, metabolic reprogramming). Transcriptomic profiles of breast cancer patients (cohort GSE20194,n=255, Gene Expression Omnibus database) were analysed with the Nexus Expression 3.0 software (BioDiscovery). The gene expression profiles of the lowest 14-3-3σ quartile were compared with those of the highest 14-3-3σ quartile and matched with corresponding biological processes and cancer hallmarks. A Circos map (circos.ca) was used to display the biological processes and cancer hallmarks that were upregulated on 14-3-3σ downregulation. The size of cancer hallmarks’ symbols indicated the magnitude of their upregulation on 14-3-3σ silencing. The bar graph on the upper right corner shows a significant increase in cancer energy metabolism when 14-3-3σ expression is downregulated. Enrichment scores were calculated based on transcriptomic analysis using the Nexus Expression 3.0 programme (BioDiscovery). Details about transcriptomic changes associated with 14-3-3σ downregulation are described inSupplementary Fig. 1 and 2. (c) Low 14-3-3σ expression is associated with increased oncogene expression and reduced levels of tumour suppressors. This Venn diagram highlights genes and biological processes with significantly changed expression when 14-3-3σ is downregulated in breast cancer patients’ tumours (cohort GSE20194,n=255, Gene Expression Omnibus database). (d) High 14-3-3σ expression is accompanied by a decrease in18FDG uptake by human breast tumours. PET scan data and gene expression profiles of patients’ breast tumours (collected at MDACC) are combined in this analysis to study the impact of 14-3-3σ on tumour glucose uptake in patients. Student'sttest. Average±95% confidence interval (CI). (e,f) Gene Set Enrichment Analysis (GSEA, Broad Institute) of breast cancer patients showed upregulation of metabolic genes in breast tumours that expressed a low level of 14-3-3σ compared with breast tumours with high 14-3-3σ expression. 1a , Supplementary Table 1 ). Bioinformatics analysis revealed marked increases in major cancer hallmarks and corresponding biological processes when 14-3-3σ was downregulated ( Fig. 1b , Supplementary Figs 1 and 2 ). 14-3-3σ downregulation in breast cancer was correlated with deregulation of cancer hallmarks, especially, deregulated cellular energetics, genomic instability, sustained proliferative signalling and resistance to cell death as illustrated by a Circos map ( Fig. 1b ). Deregulation of cellular energetics (large size of symbol) and genome instability were among the cancer hallmarks most enhanced on 14-3-3σ silencing. These observations suggest that 14-3-3σ could have broad control of tumorigenesis. Notably, elevations in genes associated with deregulation of cellular energetics (that is, glucose uptake, glycolysis, glutaminolysis, energy production and mitochondrial biogenesis) were among the most significant changes in tumour gene expression profiles associated with 14-3-3σ downregulation ( Fig. 1b,c , Supplementary Fig. 3 ). Accordingly, breast cancer patients whose tumours expressed low levels of 14-3-3σ had higher uptake of [ 18 F]fluorodeoxyglucose ( 18 FDG), indicating that loss of 14-3-3σ increases tumour glucose import ( Fig. 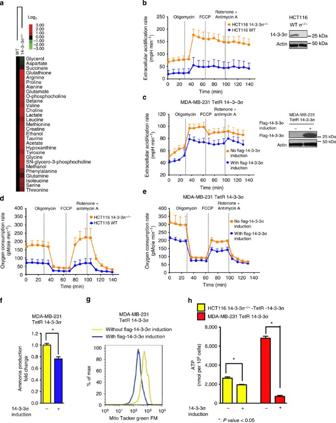Figure 2: 14-3-3σ inhibits cancer metabolic reprogramming. (a) The broad suppressive impact of 14-3-3σ on cancer metabolism. NMR was used to measure the concentrations of important metabolites in HCT116 14-3-3σ+/+(WT), HCT116 14-3-3σ−/−. (b) 14-3-3σ decreased the ECAR of HCT116in vitro.ECARs were measured by a Seahorse Extracellular Efflux Analyzer XF96 (XF96). Average±s.d.,n=3,P<0.05. (c) 14-3-3σ reduced the ECAR of MDA-MB-231in vitro. ECARs were measured by XF96. Average±s.d.,n=3,P<0.05. (d) 14-3-3σ inhibited the OCR of HCT116in vitro.OCRs were measured by XF96. Average±s.d.,n=3, Student’st-test,*P<0.05. (e) 14-3-3σ diminished the OCR of MDA-MB-231in vitro. OCRs were measured by XF96. Average±s.d.,n=3, Student’st-test,*P<0.05. (f) 14-3-3σ inhibited cancer glutaminolysis as measured using ammonia production assays. Cellular lysates of MDA-MB-231 TetR 14-3-3σ cells were collected to measure the ammonia production rate using an ammonia production kit (Sigma-Aldrich). Average±s.d.,n=3, Student’st-test,*P<0.05. (g) 14-3-3σ decreased cancer mitochondrial mass of MDA-MB-231in vitro. MDA-MB-231 TetR 14-3-3σ cells were stained with Mitochondria Tracker Green FM (Molecular Probes, Invitrogen), which stains functional mitochondria. Mitochondrial Tracker Green FM signals were analysed using a BD Biosciences FACS Canto flow cytometer. The FlowJo X software was used to build Mitochondrial Tracker Green FM histograms. Noninduced MDA-MB-231 TetR 14-3-3σ cells were used as a control. (h) Induction of 14-3-3σ expression decreased ATP concentrations in the colorectal cancer cell line HCT116 and the triple-negative breast cancer cell line MDA-MB-231in vitro. HCT116 14-3-3σ−/−TetR 14-3-3σ and MDA-MB-231 TetR 14-3-3σ cancer cells were grown in doxycycline-containing medium (5 ng ml−1) for inducing Flag-14-3-3σ expression for 3 days. Noninduced cells were used as a control. Cell lysates from HCT116 14-3-3σ−/−TetR 14-3-3σ cells and MDA-MB-231 TetR 14-3-3σ cells were collected for measuring ATP concentration using an ATP Bioluminescence CLS II kit (Roche) and a luminometer (Biotek). Average±95% CI,n=3, analysis of variance (ANOVA),*P<0.05. 1d , Supplementary Table 2 ). Likewise, 14-3-3σ silencing was correlated with elevated expression of glycolytic and glutaminolytic genes in breast tumours ( Fig. 1e,f ). These data suggest that the regulatory role of 14-3-3σ in tumorigenesis may include inhibiting metabolic reprogramming and other important cancer hallmarks. Figure 1: The clinical relevance of 14-3-3σ in breast cancer and tumour metabolic reprogramming. ( a ) High 14-3-3σ expression was associated with prolonged breast cancer patients’ survival. 14-3-3σ protein expression levels in breast cancer patients at MD Anderson Cancer Center were evaluated using immunohistochemistry staining and matched with clinical data. 14-3-3σ protein expression in normal breast tissues was used as a reference to stratify patients. Log-rank test. ( b ) Downregulation of 14-3-3σ is associated with upregulation of major cancer hallmarks especially deregulation of cellular energetics (that is, metabolic reprogramming). Transcriptomic profiles of breast cancer patients (cohort GSE20194, n =255, Gene Expression Omnibus database) were analysed with the Nexus Expression 3.0 software (BioDiscovery). The gene expression profiles of the lowest 14-3-3σ quartile were compared with those of the highest 14-3-3σ quartile and matched with corresponding biological processes and cancer hallmarks. A Circos map (circos.ca) was used to display the biological processes and cancer hallmarks that were upregulated on 14-3-3σ downregulation. The size of cancer hallmarks’ symbols indicated the magnitude of their upregulation on 14-3-3σ silencing. The bar graph on the upper right corner shows a significant increase in cancer energy metabolism when 14-3-3σ expression is downregulated. Enrichment scores were calculated based on transcriptomic analysis using the Nexus Expression 3.0 programme (BioDiscovery). Details about transcriptomic changes associated with 14-3-3σ downregulation are described in Supplementary Fig. 1 and 2 . ( c ) Low 14-3-3σ expression is associated with increased oncogene expression and reduced levels of tumour suppressors. This Venn diagram highlights genes and biological processes with significantly changed expression when 14-3-3σ is downregulated in breast cancer patients’ tumours (cohort GSE20194, n =255, Gene Expression Omnibus database). ( d ) High 14-3-3σ expression is accompanied by a decrease in 18 FDG uptake by human breast tumours. PET scan data and gene expression profiles of patients’ breast tumours (collected at MDACC) are combined in this analysis to study the impact of 14-3-3σ on tumour glucose uptake in patients. Student's t test. Average±95% confidence interval (CI). ( e,f ) Gene Set Enrichment Analysis (GSEA, Broad Institute) of breast cancer patients showed upregulation of metabolic genes in breast tumours that expressed a low level of 14-3-3σ compared with breast tumours with high 14-3-3σ expression. Full size image 14-3-3σ reduces glucose uptake and mitochondrial mass To elucidate the impact of 14-3-3σ on cancer metabolism, we analysed tumour metabolomes using NMR. We noticed that deletion of 14-3-3σ from HCT116 colorectal carcinoma cells remarkably accelerated their metabolism ( Fig. 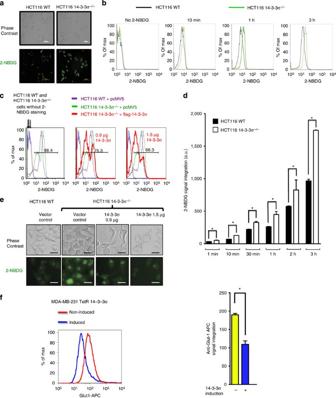Figure 3: 14-3-3σ reduces glucose uptake of colorectal and breast cancer cells. (a) Microscopic pictures show that loss of 14-3-3σ in HCT116 resulted in marked enhancement of glucose uptake. HCT116 WT (14-3-3σ+/+) and HCT116 14-3-3σ−/−cells were incubated with 2-NBDG, a green fluorescent glucose analogue that is commonly used to measure glucose uptake. 2-NBDG signals were captured using fluorescence microscopy. (b) Flow cytometry analysis indicates a significant increase in glucose uptake of 14-3-3σ-deficient cancer cells. In this experiment, HCT116 WT and HCT116 14-3-3σ−/−cells were incubated with 2-NBDG for the indicated times. 2-NBDG signals were quantified using flow cytometry. Our data point out a considerable enhancement of glucose-import activity in cancer cells on 14-3-3σ suppression. (c) Restoring 14-3-3σ expression in 14-3-3σ-deficient cells decreased glucose uptake in a dose-dependent manner. HCT116 14-3-3σ−/−cells were transfected with increasing amounts of pCMV5-Flag-14-3-3σ. 2-NBDG signals were quantified using a flow cytometer as inb. (d) Bar graph and statistical analysis of data shown inc. Data represent means±95% CI. ANOVA,*P<0.05. (e) Representative pictures from a fluorescence microscope for the experiment inc. Scale bar, 50 μm. Forced expression of 14-3-3σ in 14-3-3σ-null cancer cells reduced glucose uptake. (f) Induced 14-3-3σ decreased the expression of glucose transporter Glut1 on the cell membrane surface. Induced and noninduced cells were stained with specific anti-Glut1 antibodies conjugated with allophycocyanin (APC) fluorophore and analysed using flow cytometry. Bars represent means±95% CI; Student’st-test, *P<0.05. 2a , Supplementary Table 3 ). When 14-3-3σ expression was restored by adenoviral infection, metabolism and biosynthesis were largely suppressed ( Supplementary Fig. 4 , Supplementary Table 3 ). Interestingly, the lactate level was tightly controlled by 14-3-3σ. Lactate is a potent oncometabolite that accelerates tumorigenesis [30] , [31] , supports tumour survival and facilitates metastasis [2] , [3] , [4] , [7] , [8] , [13] . 14-3-3σ also regulated the concentrations of important amino acids, such as arginine, proline, alanine, valine, leucine, methionine, tyrosine, serine and threonine, and essential metabolic precursors, such as phosphocholine, taurine and hypoxanthine ( Fig. 2a , Supplementary Table 3 ). These metabolites are indispensable building blocks for tumour biosynthesis, growth and proliferation [32] . Figure 2: 14-3-3σ inhibits cancer metabolic reprogramming. ( a ) The broad suppressive impact of 14-3-3σ on cancer metabolism. NMR was used to measure the concentrations of important metabolites in HCT116 14-3-3σ +/+ (WT), HCT116 14-3-3σ −/− . ( b ) 14-3-3σ decreased the ECAR of HCT116 in vitro. ECARs were measured by a Seahorse Extracellular Efflux Analyzer XF96 (XF96). Average±s.d., n =3, P <0.05. ( c ) 14-3-3σ reduced the ECAR of MDA-MB-231 in vitro . ECARs were measured by XF96. Average±s.d., n =3, P <0.05. ( d ) 14-3-3σ inhibited the OCR of HCT116 in vitro. OCRs were measured by XF96. Average±s.d., n =3, Student’s t -test,* P <0.05. ( e ) 14-3-3σ diminished the OCR of MDA-MB-231 in vitro . OCRs were measured by XF96. Average±s.d., n =3, Student’s t -test,* P <0.05. ( f ) 14-3-3σ inhibited cancer glutaminolysis as measured using ammonia production assays. Cellular lysates of MDA-MB-231 TetR 14-3-3σ cells were collected to measure the ammonia production rate using an ammonia production kit (Sigma-Aldrich). Average±s.d., n =3, Student’s t -test,* P <0.05. ( g ) 14-3-3σ decreased cancer mitochondrial mass of MDA-MB-231 in vitro . MDA-MB-231 TetR 14-3-3σ cells were stained with Mitochondria Tracker Green FM (Molecular Probes, Invitrogen), which stains functional mitochondria. Mitochondrial Tracker Green FM signals were analysed using a BD Biosciences FACS Canto flow cytometer. The FlowJo X software was used to build Mitochondrial Tracker Green FM histograms. Noninduced MDA-MB-231 TetR 14-3-3σ cells were used as a control. ( h ) Induction of 14-3-3σ expression decreased ATP concentrations in the colorectal cancer cell line HCT116 and the triple-negative breast cancer cell line MDA-MB-231 in vitro . HCT116 14-3-3σ −/− TetR 14-3-3σ and MDA-MB-231 TetR 14-3-3σ cancer cells were grown in doxycycline-containing medium (5 ng ml −1 ) for inducing Flag-14-3-3σ expression for 3 days. Noninduced cells were used as a control. Cell lysates from HCT116 14-3-3σ −/− TetR 14-3-3σ cells and MDA-MB-231 TetR 14-3-3σ cells were collected for measuring ATP concentration using an ATP Bioluminescence CLS II kit (Roche) and a luminometer (Biotek). Average±95% CI, n =3, analysis of variance (ANOVA),* P <0.05. Full size image We also showed that deletion and knockdown of 14-3-3σ increased extracellular acidification rate (ECAR), an indicator of glycolysis, in colorectal and breast cancer cells ( Fig. 2b , Supplementary Fig 5a ). 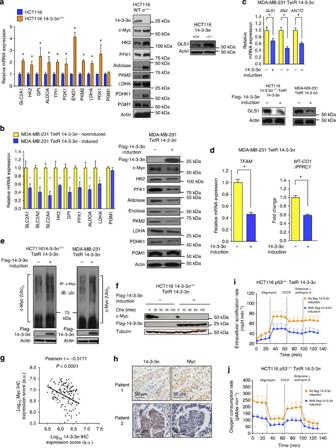Figure 5: 14-3-3σ inhibits cancer metabolism by promoting Myc degradation. (a) Loss of 14-3-3σ upregulated Myc-induced glycolytic genes. The expression of glycolytic genes in HCT116 WT (14-3-3σ+/+) and HCT116 14-3-3σ−/−cells were measured using real-time PCR (left panel). Average±95% CI,n=4, ANOVA,*P<0.05. Western blot analysis was performed using the indicated antibodies (right panel). (b) 14-3-3σ downregulated Myc-induced glycolytic genes. The mRNA expression levels of glycolytic genes were compared between indicated cells using real-time PCR (left panel). Average±95% CI,n=3, ANOVA,*P<0.05. Western blot analysis was performed using the indicated antibodies (right panel). (c) 14-3-3σ reduced expression of Myc-induced glutaminolytic genes. Real-time PCR and western blot analyses were used to compare the expression of Myc-induced glutaminolytic genes at mRNA and protein levels. Average±95% CI,n=3, ANOVA,*P<0.05. (d) 14-3-3σ suppressedTFAMexpression and reducedMT-CO1/PPRC1ratioin vitro.TFAMis an important Myc-induced mitochondrial transcription factor.MT-CO1is a mitochondrial gene encoding cytochromecoxidase.PPRC1, peroxisome proliferator-activated receptor gamma, co-activator-related 1, is a gene of nuclear DNA. Average±95% CI,n=3, Student’st-test, *P<0.05. (e) 14-3-3σ increased Myc ubiquitination. Indicated cells were treated with Doxycycline to induce Flag-14-3-3σ expression (+). Noninduced cells were used as a control (−). Cell lysates were immunoprecipitated with anti-Myc antibodies and immunoblotted with antiubiquitin antibodies. (f) 14-3-3σ shortened Myc half-life. Flag-14-3-3σ was induced by doxycycline in indicated cells. Cells were treated with 200 μg ml−1Cycloheximide (Chx) for the indicated times. Cell lysates are immunoblotted with indicated antibodies. (g) 14-3-3σ expression was inversely correlated with the Myc level in 145 patients’ breast tumours. 14-3-3σ and Myc protein expression levels were quantified from immunohistochemistry (IHC) staining of breast cancer patients’ tissue microarrays collected at MDACC. Correlation analysis and graph was built using the GraphPad Prism software. (h) Representative immunohistochemistry images ofgshowing the negative correlation between 14-3-3σ and Myc protein expression in breast cancer. (i) 14-3-3σ diminished the ECARs of HCT116 p53−/−in vitro. ECARs were measured by XF96. Average±s.d.,n=4,P<0.05. (j) 14-3-3σ diminished the OCRs of the p53-deficient colon cancer cell line HCT116 p53−/−in vitro. OCRs were measured by XF96. Average±s.d.,n=4,P<0.05. In contrast, induced expression of 14-3-3σ reduced ECAR ( Fig. 2c , Supplementary Fig. 5b ). 14-3-3σ also suppressed mitochondrial respiration as indicated by the oxygen consumption rate (OCR; Fig. 2d,e , Supplementary Fig. 6 ). In the OCR assay, oligomycin, which prevents ATP synthesis, is added to inhibit oxygen consumption. However, oxygen consumption can be stimulated again when oxidative phosphorylation is uncoupled by addition of FCCP (p-trifluoromethoxy carbonyl cyanide phenylhydrazone), which destroys the mitochondrial membrane potential and causes a short circuit in the respiratory chain. Following this, oxygen consumption can be completely stopped when rotenone (inhibitor of mitochondrial complex I) and antimycin A (inhibitor of mitochondrial complex III) are added to block the electron transport chain. Other independent biochemical assays additionally demonstrated that 14-3-3σ inhibited glucose consumption, lactate production and glucose uptake of cancer cells ( Fig. 3 , Supplementary Figs 7 and 8 ). Furthermore, 14-3-3σ decreased glutaminolysis, mitochondrial mass and energy production in breast, colorectal and lung cancer cells ( Figs 2f–h and 4 , Supplementary Fig. 9 ). Thus, our data show that 14-3-3σ potently antagonizes tumour metabolic reprogramming, an important cancer hallmark. Figure 3: 14-3-3σ reduces glucose uptake of colorectal and breast cancer cells. ( a ) Microscopic pictures show that loss of 14-3-3σ in HCT116 resulted in marked enhancement of glucose uptake. HCT116 WT (14-3-3σ +/+ ) and HCT116 14-3-3σ −/− cells were incubated with 2-NBDG, a green fluorescent glucose analogue that is commonly used to measure glucose uptake. 2-NBDG signals were captured using fluorescence microscopy. ( b ) Flow cytometry analysis indicates a significant increase in glucose uptake of 14-3-3σ-deficient cancer cells. In this experiment, HCT116 WT and HCT116 14-3-3σ −/− cells were incubated with 2-NBDG for the indicated times. 2-NBDG signals were quantified using flow cytometry. Our data point out a considerable enhancement of glucose-import activity in cancer cells on 14-3-3σ suppression. ( c ) Restoring 14-3-3σ expression in 14-3-3σ-deficient cells decreased glucose uptake in a dose-dependent manner. HCT116 14-3-3σ −/− cells were transfected with increasing amounts of pCMV5-Flag-14-3-3σ. 2-NBDG signals were quantified using a flow cytometer as in b . ( d ) Bar graph and statistical analysis of data shown in c . Data represent means±95% CI. ANOVA,* P <0.05. ( e ) Representative pictures from a fluorescence microscope for the experiment in c . Scale bar, 50 μm. Forced expression of 14-3-3σ in 14-3-3σ-null cancer cells reduced glucose uptake. ( f ) Induced 14-3-3σ decreased the expression of glucose transporter Glut1 on the cell membrane surface. Induced and noninduced cells were stained with specific anti-Glut1 antibodies conjugated with allophycocyanin (APC) fluorophore and analysed using flow cytometry. 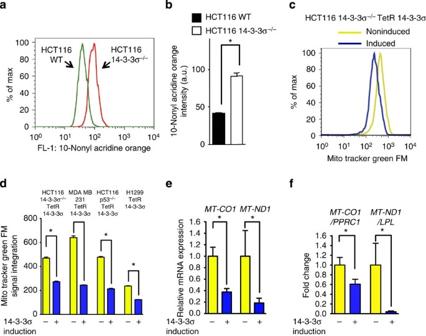Bars represent means±95% CI; Student’s t -test, * P <0.05. Figure 4: 14-3-3σ reduces mitochondrial mass of cancer cells. (a,b) 14-3-3σ decreased mitochondrial mass of HCT116 colorectal carcinoma cells. HCT116 14-3-3σ+/+(WT) and HCT116 14-3-3σ−/−cells were stained with 10-nonyl acridine orange (10-NAO; Molecular Probes, Invitrogen). 10-NAO is an orange dye associated with mitochondrial cardiolipin. Therefore, 10-NAO is frequently used to evaluate total mitochondrial mass. In this experiment, 10-NAO signal was quantified using flow cytometry and is displayed as a histogram (a) and a bar graph (b). Bars represent average±95% CI; Student’st-test, *P<0.05. (c) Restoring 14-3-3σ expression led to a significant decline in mitochondrial mass in HCT116 14-3-3σ−/−cells. Flag-14-3-3σ expression was induced in HCT116 14-3-3σ−/−cells. Noninduced cells were used as a control. All cells were stained with MitoTracker Green FM, a green fluorescent dye used to quantify functional mitochondrial mass. MitoTracker Green FM signals were analysed using flow cytometry. (d) Bar graph of data fromcshow the suppressive effect of 14-3-3σ on mitochondrial mass of multiple cancer cell lines. Bars represent means±95% CI; Student’st-test, *P<0.05. Notably, the inhibitory impact of 14-3-3σ on mitochondrial biogenesis was also observed in p53-deficient cancer cells (HCT116 p53−/−and H1299). (e) 14-3-3σ decreased mitochondrial gene expression. Flag-14-3-3σ expression was induced in HCT116 14-3-3σ−/−TetR 14-3-3σ and MDA-MB-231 TetR 14-3-3σ cells. Real-time PCR was performed using specific primers for the mitochondrial genesMT-CO1andMT-ND1. Bars represent average±95% CI; Student’st-test, *P<0.05. (f) 14-3-3σ diminished mitochondrial DNA copy number. Flag-14-3-3σ expression was induced in HCT116 14-3-3σ−/−TetR 14-3-3σ cells. Noninduced cells were used as a control. The expression ratios ofMT-CO1/PPRC1andMT-ND1/LPLwere quantitated by using real-time PCR. Bars represent average±95% CI; Student’st-test, *P<0.05. WhileMT-CO1andMT-ND1genes are located in mitochondrial DNA,PPRC1andLPL1are encoded in the nucleus. Therefore, reduction ofMT-CO1/PPRC1andMT-ND1/LPLratios reflects a decrease in mitochondrial DNA content or mitochondrial number because of 14-3-3σ. Full size image Figure 4: 14-3-3σ reduces mitochondrial mass of cancer cells. ( a,b ) 14-3-3σ decreased mitochondrial mass of HCT116 colorectal carcinoma cells. HCT116 14-3-3σ +/+ (WT) and HCT116 14-3-3σ −/− cells were stained with 10-nonyl acridine orange (10-NAO; Molecular Probes, Invitrogen). 10-NAO is an orange dye associated with mitochondrial cardiolipin. Therefore, 10-NAO is frequently used to evaluate total mitochondrial mass. In this experiment, 10-NAO signal was quantified using flow cytometry and is displayed as a histogram ( a ) and a bar graph ( b ). Bars represent average±95% CI; Student’s t -test, * P <0.05. ( c ) Restoring 14-3-3σ expression led to a significant decline in mitochondrial mass in HCT116 14-3-3σ −/− cells. Flag-14-3-3σ expression was induced in HCT116 14-3-3σ −/− cells. Noninduced cells were used as a control. All cells were stained with MitoTracker Green FM, a green fluorescent dye used to quantify functional mitochondrial mass. MitoTracker Green FM signals were analysed using flow cytometry. ( d ) Bar graph of data from c show the suppressive effect of 14-3-3σ on mitochondrial mass of multiple cancer cell lines. Bars represent means±95% CI; Student’s t -test, * P <0.05. Notably, the inhibitory impact of 14-3-3σ on mitochondrial biogenesis was also observed in p53-deficient cancer cells (HCT116 p53 −/− and H1299). ( e ) 14-3-3σ decreased mitochondrial gene expression. Flag-14-3-3σ expression was induced in HCT116 14-3-3σ −/− TetR 14-3-3σ and MDA-MB-231 TetR 14-3-3σ cells. Real-time PCR was performed using specific primers for the mitochondrial genes MT-CO1 and MT-ND1 . Bars represent average±95% CI; Student’s t -test, * P <0.05. ( f ) 14-3-3σ diminished mitochondrial DNA copy number. Flag-14-3-3σ expression was induced in HCT116 14-3-3σ −/− TetR 14-3-3σ cells. Noninduced cells were used as a control. The expression ratios of MT-CO1/PPRC1 and MT-ND1/LPL were quantitated by using real-time PCR. Bars represent average±95% CI; Student’s t -test, * P <0.05. While MT-CO1 and MT-ND1 genes are located in mitochondrial DNA, PPRC1 and LPL1 are encoded in the nucleus. Therefore, reduction of MT-CO1/PPRC1 and MT-ND1/LPL ratios reflects a decrease in mitochondrial DNA content or mitochondrial number because of 14-3-3σ. Full size image 14-3-3σ diminishes Myc target genes in metabolism To decipher how 14-3-3σ controls cancer metabolism, we analysed the expression of the key cancer metabolic genes and regulators in cancer cells. We observed that loss and knockdown of 14-3-3σ upregulated many glycolytic genes, especially those induced by Myc ( Fig. 5a , Supplementary Fig. 10 ). Notably, the Myc protein level increased in 14-3-3σ-deficient and 14-3-3σ-knockdown cancer cells, while restoration of 14-3-3σ expression downregulated Myc and its glycolytic target genes ( Fig. 5b ). Likewise, 14-3-3σ downregulated Myc target genes involved in glutaminolysis, such as Gls , Slc38a5 (Sn2) and Slc1a5 (Asct2 ; Fig. 5c , Supplementary Fig. 11 ). 14-3-3σ also decreased the expression of Tfam , a Myc-transactivated mitochondrial transcription factor that is required for mitochondrial biogenesis ( Fig. 5d , Supplementary Fig. 12 ) [12] . The observation that 14-3-3σ reduced mitochondrial biogenesis is significant because mitochondria are not only the energy generators but also the nexus of many metabolic/biosynthetic pathways that are vital for tumours [33] , [34] . Figure 5: 14-3-3σ inhibits cancer metabolism by promoting Myc degradation. ( a ) Loss of 14-3-3σ upregulated Myc-induced glycolytic genes. The expression of glycolytic genes in HCT116 WT (14-3-3σ +/+ ) and HCT116 14-3-3σ −/− cells were measured using real-time PCR (left panel). Average±95% CI, n =4, ANOVA,* P <0.05. Western blot analysis was performed using the indicated antibodies (right panel). ( b ) 14-3-3σ downregulated Myc-induced glycolytic genes. The mRNA expression levels of glycolytic genes were compared between indicated cells using real-time PCR (left panel). Average±95% CI, n =3, ANOVA,* P <0.05. Western blot analysis was performed using the indicated antibodies (right panel). ( c ) 14-3-3σ reduced expression of Myc-induced glutaminolytic genes. Real-time PCR and western blot analyses were used to compare the expression of Myc-induced glutaminolytic genes at mRNA and protein levels. Average±95% CI, n =3, ANOVA,* P <0.05. ( d ) 14-3-3σ suppressed TFAM expression and reduced MT-CO1/PPRC1 ratio in vitro . TFAM is an important Myc-induced mitochondrial transcription factor. MT-CO1 is a mitochondrial gene encoding cytochrome c oxidase. PPRC1 , peroxisome proliferator-activated receptor gamma, co-activator-related 1, is a gene of nuclear DNA. Average±95% CI, n =3, Student’s t -test, * P <0.05. ( e ) 14-3-3σ increased Myc ubiquitination. Indicated cells were treated with Doxycycline to induce Flag-14-3-3σ expression (+). Noninduced cells were used as a control (−). Cell lysates were immunoprecipitated with anti-Myc antibodies and immunoblotted with antiubiquitin antibodies. ( f ) 14-3-3σ shortened Myc half-life. Flag-14-3-3σ was induced by doxycycline in indicated cells. Cells were treated with 200 μg ml −1 Cycloheximide (Chx) for the indicated times. Cell lysates are immunoblotted with indicated antibodies. ( g ) 14-3-3σ expression was inversely correlated with the Myc level in 145 patients’ breast tumours. 14-3-3σ and Myc protein expression levels were quantified from immunohistochemistry (IHC) staining of breast cancer patients’ tissue microarrays collected at MDACC. Correlation analysis and graph was built using the GraphPad Prism software. ( h ) Representative immunohistochemistry images of g showing the negative correlation between 14-3-3σ and Myc protein expression in breast cancer. ( i ) 14-3-3σ diminished the ECARs of HCT116 p53 −/− in vitro . ECARs were measured by XF96. Average±s.d., n =4, P <0.05. ( j ) 14-3-3σ diminished the OCRs of the p53-deficient colon cancer cell line HCT116 p53 −/− in vitro . OCRs were measured by XF96. Average±s.d., n =4, P <0.05. Full size image In addition, we found that 14-3-3σ promoted Myc polyubiquitination, shortened Myc half-life and suppressed Myc transcriptional activity ( Fig. 5e,f , Supplementary Fig. 13 ). Analysis of breast tumours from patients showed an inverse correlation between Myc and 14-3-3σ protein levels ( Fig. 5g,h ). Myc knockdown in cancer cells by lentiviral short hairpin RNA (shRNA) revealed that targeting Myc is a major mechanism by which 14-3-3σ controls cancer metabolism ( Fig. 6 ). Moreover, 14-3-3σ effectively inhibited cancer metabolic reprogramming even in the absence of p53 ( Figs 5i,j and 7 ). This finding emphasizes the therapeutic potential of 14-3-3σ because p53 is frequently mutated or inactivated, especially in aggressive and metastatic tumours. Thus, 14-3-3σ efficiently inhibits tumour metabolism by promoting Myc degradation and functions well in p53-deficient cancer cells. 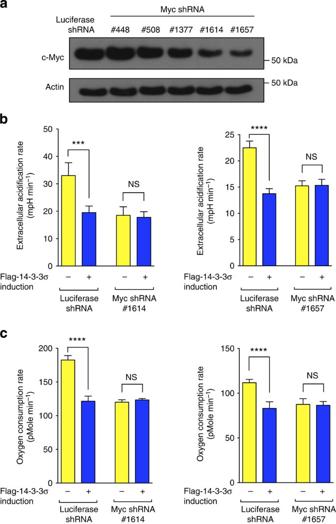Figure 6: Targeting c-Myc is a mechanism by which 14-3-3σ suppresses cancer metabolic reprogramming. (a) c-Myc expression was knocked down in MDA-MB-231 TetR 14-3-3σ breast cancer cells. (b,c) c-Myc knockdown hindered 14-3-3σ-mediated suppression of cancer metabolic reprogramming. MDA-MB-231 TetR 14-3-3σ cells infected with luciferase shRNA, c-Myc shRNA #1614 or c-Myc shRNA #1657 were treated with doxycycline to induce Flag-14-3-3σ expression (+). Noninduced cells were used as a control (−). ECAR and OCR were measured as previously described. Bars represent means±95% CI; Student’st-test, *P<0.05. Figure 6: Targeting c-Myc is a mechanism by which 14-3-3σ suppresses cancer metabolic reprogramming. ( a ) c-Myc expression was knocked down in MDA-MB-231 TetR 14-3-3σ breast cancer cells. ( b,c ) c-Myc knockdown hindered 14-3-3σ-mediated suppression of cancer metabolic reprogramming. MDA-MB-231 TetR 14-3-3σ cells infected with luciferase shRNA, c-Myc shRNA #1614 or c-Myc shRNA #1657 were treated with doxycycline to induce Flag-14-3-3σ expression (+). Noninduced cells were used as a control (−). ECAR and OCR were measured as previously described. Bars represent means±95% CI; Student’s t -test, * P <0.05. 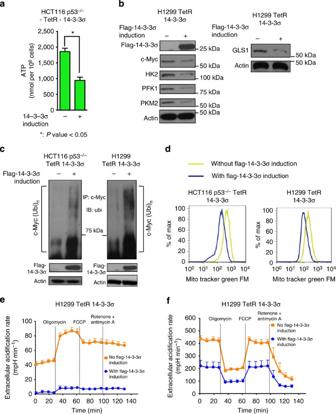Figure 7: 14-3-3σ effectively suppresses metabolic reprogramming in p53-deficient colorectal and lung cancer cells. (a) 14-3-3σ expression decreased energy production in p53-deficient colorectal carcinoma cells. ATP measurements were shown. Bars represent means±95% CI; Student’st-test, *P<0.05. (b) 14-3-3σ reduced expression of c-Myc as well as c-Myc glycolytic and glutaminolytic targets in p53-null H1299 lung cancer cells. Flag-14-3-3σ expression was induced in the cells. c-Myc, HK2, PFK1, PKM2 and GLS1 protein levels of induced and noninduced H1299 cells were compared. (c) 14-3-3σ promoted c-Myc polyubiquitination in p53-deficient cancer cells. Flag-14-3-3σ expression was induced in indicated cells (+). Noninduced cells were used as a control (−). Cell lysates were immunoprecipitated with anti-c-Myc antibodies and immunoblotted with antiubiquitin (ubi) antibodies. (d) Induction of 14-3-3σ expression reduced mitochondrial mass of p53-null cancer cells. Mitochondria of HCT116 p53−/−TetR 14-3-3σ and H1299 TetR 14-3-3σ cells were stained with MitoTracker Green FM. (e) 14-3-3σ reduced ECAR of p53-null H1299 cells. ECAR, which reflects glycolytic activity, was measured in induced and noninduced H1299 TetR 14-3-3σ cells. (f) 14-3-3σ suppressed oxygen consumption and mitochondrial respiration in p53-deficient cells. Oxygen consumption and mitochondrial respiration of induced and noninduced H1299 TetR 14-3-3σ were measured. Full size image Figure 7: 14-3-3σ effectively suppresses metabolic reprogramming in p53-deficient colorectal and lung cancer cells. ( a ) 14-3-3σ expression decreased energy production in p53-deficient colorectal carcinoma cells. ATP measurements were shown. Bars represent means±95% CI; Student’s t -test, * P <0.05. ( b ) 14-3-3σ reduced expression of c-Myc as well as c-Myc glycolytic and glutaminolytic targets in p53-null H1299 lung cancer cells. Flag-14-3-3σ expression was induced in the cells. c-Myc, HK2, PFK1, PKM2 and GLS1 protein levels of induced and noninduced H1299 cells were compared. ( c ) 14-3-3σ promoted c-Myc polyubiquitination in p53-deficient cancer cells. Flag-14-3-3σ expression was induced in indicated cells (+). Noninduced cells were used as a control (−). Cell lysates were immunoprecipitated with anti-c-Myc antibodies and immunoblotted with antiubiquitin (ubi) antibodies. ( d ) Induction of 14-3-3σ expression reduced mitochondrial mass of p53-null cancer cells. Mitochondria of HCT116 p53 −/− TetR 14-3-3σ and H1299 TetR 14-3-3σ cells were stained with MitoTracker Green FM. ( e ) 14-3-3σ reduced ECAR of p53-null H1299 cells. ECAR, which reflects glycolytic activity, was measured in induced and noninduced H1299 TetR 14-3-3σ cells. ( f ) 14-3-3σ suppressed oxygen consumption and mitochondrial respiration in p53-deficient cells. Oxygen consumption and mitochondrial respiration of induced and noninduced H1299 TetR 14-3-3σ were measured. Full size image 14-3-3σ is also regulating metabolism under hypoxia Interestingly, our data showed that 14-3-3σ also decreased ECARs of HCT116 and MDA-MB-231 cells in hypoxia ( Fig. 8a,b ). Loss and knockdown of 14-3-3σ promoted glycolytic gene expression of HCT116 cells cultured under a hypoxic condition ( Fig. 8c,d ). These observations further highlight the potential of 14-3-3σ in regulating cancer metabolism. We additionally observed that HCT116 14-3-3σ −/− proliferated much slower when glucose was replaced by galactose in culture medium ( Supplementary Fig. 14 ). Loss of 14-3-3σ also rendered HCT116 cells addicted to glutaminolysis, a commonly seen phenomenon in cancer cells that have high levels of Myc expression ( Supplementary Fig. 15 ). Furthermore, we noticed that induction of Flag-14-3-3σ expression significantly induced cell death of HCT116 14-3-3σ colon cancer cells, MDA-MB-231 metastatic breast cancer cells and H1299 lung cancer cells ( Supplementary Fig. 16 ), which indicates the potential of 14-3-3σ in anticancer therapies. 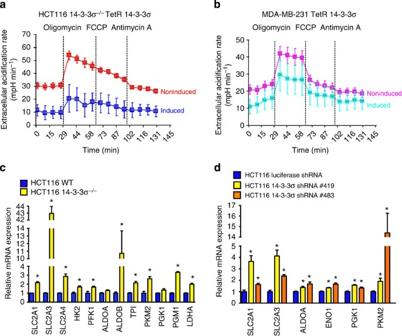Figure 8: 14-3-3σ is involved in metabolic regulation under hypoxic condition. (a,b) Induction of Flag-14-3-3σ expression in HCT116 14-3-3σ−/−and MDA-MB-231 cells decreases ECAR in hypoxia. HCT116 14-3-3σ−/−TetR 14-3-3σ cells and MDA-MB-231 TetR 14-3-3σ cells were grown in a hypoxic chamber for 48 h. Flag-14-3-3σ expression was induced for 48 h by adding doxycycline to the culture medium. Noninduced cells were used as a control. ECARs were measured using a Seahorse Extracellular Flux analyzer XF24 (Seahorse Biosciences).n=3; Average±s.d. Student’st-test, *P<0.05. (c,d) Loss or knockdown of 14-3-3σ results in an increase in glycolytic gene mRNA expression in hypoxia. HCT116 WT (14-3-3σ+/+), HCT116 14-3-3σ−/−, HCT116 Luciferase shRNA, HCT116 14-3-3σ shRNA #419 and HCT116 14-3-3σ shRNA #483 cells were grown in a hypoxic chamber for 48 h. Total mRNA of these cells were extracted and converted to cDNA for real-time PCR reactions with specific primers as indicated above.n=4; average±95% CI; ANOVA,*P<0.05. Figure 8: 14-3-3σ is involved in metabolic regulation under hypoxic condition. ( a,b ) Induction of Flag-14-3-3σ expression in HCT116 14-3-3σ −/− and MDA-MB-231 cells decreases ECAR in hypoxia. HCT116 14-3-3σ −/− TetR 14-3-3σ cells and MDA-MB-231 TetR 14-3-3σ cells were grown in a hypoxic chamber for 48 h. Flag-14-3-3σ expression was induced for 48 h by adding doxycycline to the culture medium. Noninduced cells were used as a control. ECARs were measured using a Seahorse Extracellular Flux analyzer XF24 (Seahorse Biosciences). n =3; Average±s.d. Student’s t -test, * P <0.05. ( c,d ) Loss or knockdown of 14-3-3σ results in an increase in glycolytic gene mRNA expression in hypoxia. HCT116 WT (14-3-3σ +/+ ), HCT116 14-3-3σ −/− , HCT116 Luciferase shRNA, HCT116 14-3-3σ shRNA #419 and HCT116 14-3-3σ shRNA #483 cells were grown in a hypoxic chamber for 48 h. Total mRNA of these cells were extracted and converted to cDNA for real-time PCR reactions with specific primers as indicated above. n =4; average±95% CI; ANOVA,* P <0.05. Full size image 14-3-3σ mitigates tumour metabolic reprogramming in vivo To validate the function of 14-3-3σ in vivo , we established an orthotopic xenograft mouse model using MDA-MB-231 cells carrying an inducible tet-On 14-3-3σ expression system ( Supplementary Fig. 17 ). The induction of 14-3-3σ reduced cell proliferation and cell viability ( Supplementary Fig. 17 ). MDA-MB-231 is a highly metastatic breast cancer cell line that loses 14-3-3σ expression because of hypermethylation of the CpG islands of the SFN promoter area ( Supplementary Fig. 18 ). The experimental mouse group received doxycycline for 2 weeks to induce 14-3-3σ expression, while the control group received no doxycycline. We then used 18 FDG microPET scans to assess the impact of 14-3-3σ on tumour glucose uptake in vivo . Our data show that restoring 14-3-3σ expression caused a 50% reduction in glucose uptake by the xenograft tumours ( Fig. 9a ). This observation is interesting because glucose is a major source of energy and nutrients for cancer cells [1] , [2] , [3] . 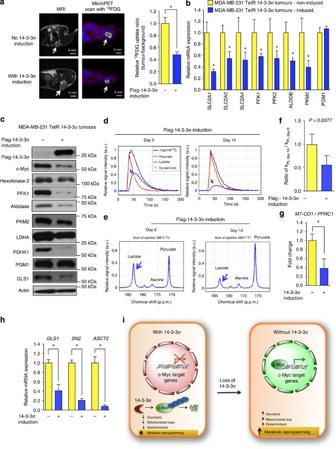Figure 9: 14-3-3σ inhibits tumour metabolic reprogrammingin vivo. (a) Doxycycline-induced Flag-14-3-3σ expression results in a remarkable decrease in18FDG uptake in MDA-MB-231 xenograft breast tumours. MDA-MB-231 TetR 14-3-3σ breast cancer cells were injected into the mammary fat pad of a female nude mouse. 14-3-3σ expression was induced by doxycycline. All mice were then imaged with Magnetic Resonance Imaging and microPET Scan. The white arrows indicate tumour location. The relative18FDG uptake ratio was calculated.n=5; average±95% CI; *P<0.05. (b) 14-3-3σ downregulated Myc-induced glycolytic genes in xenograft breast tumours. After microPET and MRI imaging, tumours were extracted from the mice. Indicated mRNA levels were measured using real-time PCR. Average±95% CI, ANOVA,*P<0.05. (c) 14-3-3σ reduced levels of Myc and Myc-induced glycolytic and glutaminolytic proteins in xenograft tumours. Cell lysates were immunoblotted with the indicated antibodies. (d) 14-3-3σ decelerated the [13C]pyruvate-to-[13C]lactate flux in MDA-MB-231 TetR 14-3-3σ xenograft tumours. The pyruvate-to-lactate flux was measured using hyperpolarized13C pyruvate tracer and MRSI, following the time course on day 0 (before Flag-14-3-3σ induction) and day 14 (after Flag-14-3-3σ induction). (e) Magnetic resonance chemical shift spectra ofdshowing Flag-14-3-3σ induction decreased13C lactate concentration in MDA-MB-231 TetR 14-3-3σ xenograft tumours. (f) Flag-14-3-3σ expression decelerates the rate constant of13C pyruvate-to-13C lactate reaction in MDA-MB-231 TetR 14-3-3σ xenograft tumours.kPLrepresents the rate constant of13C pyruvate-to-13C lactate reaction. The ratio ofkPL day 14/kPL day 0was calculated. All data are represented as average±95% CI; *P<0.05. (g) Flag-14-3-3σ induction decreasedMT-CO1/PPRC1(mitochondrial DNA/nuclear DNA) ratioin vivo. Average±95% CI; *P<0.05 (h) 14-3-3σ decreased Myc-induced glutaminolytic gene expression in MDA-MB-231 TetR 14-3-3σ xenograft tumours. Indicated mRNA levels were measured using real-time PCR. Average±95% CI, ANOVA,*P<0.05. (i) Proposed working model: when 14-3-3σ is present, it promotes Myc degradation and keeps cellular metabolism in check. As tumours evolve, 14-3-3σ is silenced by hypermethylation of its promoter area or by an increase in 14-3-3σ-targeting E3 ubiquitin ligases (for example, Efp, COP1). After escaping from 14-3-3σ-mediated regulation, Myc is stabilized and reprogrammes tumour metabolism. Restoring the function of 14-3-3σ in tumours may inhibit cancer bioenergetics and reverse cancer metabolic reprogramming. Figure 9: 14-3-3σ inhibits tumour metabolic reprogramming in vivo. ( a ) Doxycycline-induced Flag-14-3-3σ expression results in a remarkable decrease in 18 FDG uptake in MDA-MB-231 xenograft breast tumours. MDA-MB-231 TetR 14-3-3σ breast cancer cells were injected into the mammary fat pad of a female nude mouse. 14-3-3σ expression was induced by doxycycline. All mice were then imaged with Magnetic Resonance Imaging and microPET Scan. The white arrows indicate tumour location. The relative 18 FDG uptake ratio was calculated. n =5; average±95% CI; * P <0.05. ( b ) 14-3-3σ downregulated Myc-induced glycolytic genes in xenograft breast tumours. After microPET and MRI imaging, tumours were extracted from the mice. Indicated mRNA levels were measured using real-time PCR. Average±95% CI, ANOVA,* P <0.05. ( c ) 14-3-3σ reduced levels of Myc and Myc-induced glycolytic and glutaminolytic proteins in xenograft tumours. Cell lysates were immunoblotted with the indicated antibodies. ( d ) 14-3-3σ decelerated the [ 13 C]pyruvate-to-[ 13 C]lactate flux in MDA-MB-231 TetR 14-3-3σ xenograft tumours. The pyruvate-to-lactate flux was measured using hyperpolarized 13 C pyruvate tracer and MRSI, following the time course on day 0 (before Flag-14-3-3σ induction) and day 14 (after Flag-14-3-3σ induction). ( e ) Magnetic resonance chemical shift spectra of d showing Flag-14-3-3σ induction decreased 13 C lactate concentration in MDA-MB-231 TetR 14-3-3σ xenograft tumours. ( f ) Flag-14-3-3σ expression decelerates the rate constant of 13 C pyruvate-to- 13 C lactate reaction in MDA-MB-231 TetR 14-3-3σ xenograft tumours. k PL represents the rate constant of 13 C pyruvate-to- 13 C lactate reaction. The ratio of k PL day 14 / k PL day 0 was calculated. All data are represented as average±95% CI; * P <0.05. ( g ) Flag-14-3-3σ induction decreased MT-CO1/PPRC1 (mitochondrial DNA/nuclear DNA) ratio in vivo . Average±95% CI; * P <0.05 ( h ) 14-3-3σ decreased Myc-induced glutaminolytic gene expression in MDA-MB-231 TetR 14-3-3σ xenograft tumours. Indicated mRNA levels were measured using real-time PCR. Average±95% CI, ANOVA,* P <0.05. ( i ) Proposed working model: when 14-3-3σ is present, it promotes Myc degradation and keeps cellular metabolism in check. As tumours evolve, 14-3-3σ is silenced by hypermethylation of its promoter area or by an increase in 14-3-3σ-targeting E3 ubiquitin ligases (for example, Efp, COP1). After escaping from 14-3-3σ-mediated regulation, Myc is stabilized and reprogrammes tumour metabolism. Restoring the function of 14-3-3σ in tumours may inhibit cancer bioenergetics and reverse cancer metabolic reprogramming. Full size image Accordingly, induction of 14-3-3σ in these xenografts suppressed all Myc-induced target genes that are involved in glycolysis/glutaminolysis ( Fig. 9b,c ). To dynamically monitor the influence of 14-3-3σ on cancer metabolism in vivo , we employed magnetic resonance spectroscopy imaging (MRSI) and hyperpolarized [ 13 C]pyruvate tracers [35] , [36] , [37] . This metabolic imaging modality allowed us to evaluate how much and how fast the [ 13 C]pyruvate tracer was converted to lactate, alanine or acetyl-coenzyme A in real time. This is important because pyruvate-to-lactate conversion is a crucial biochemical reaction in cancer cells, especially in aggressive and metastatic tumours. By converting pyruvate to lactate, cancer cells rapidly regenerate NAD + to dramatically accelerate glycolysis, a major cancer metabolic pathway [3] , [9] . Besides, lactate is an important oncometabolite as previously mentioned [9] . Interestingly, our measurements show that after 2 weeks of 14-3-3σ induction (day 14), the [ 13 C]pyruvate-to-[ 13 C]lactate flux markedly decreased in xenograft tumours compared with control tumours (day 0; Fig. 9d ). Magnetic resonance chemical shift spectra affirmed that 14-3-3σ hindered [ 13 C]pyruvate-to-[ 13 C]lactate conversion ( Fig. 9e ). The rate constant of the [ 13 C]pyruvate-to-[ 13 C]lactate reaction in MDA-MB-231 xenograft tumours was calculated [38] and shown to be 45% lower after induction of 14-3-3σ than in the control group ( Fig. 9f ). 14-3-3σ also decreased mitochondrial DNA ( Fig. 9g , Supplementary Fig. 19 ) and glutaminolysis ( Fig. 9c,h ) in the xenografts. Moreover, 14-3-3σ increased apoptosis in xenograft tumours ( Supplementary Fig. 20 ), which could have been due to the inhibitory interference of 14-3-3σ in cancer bioenergetics and metabolism. Induction of 14-3-3σ also suppressed xenograft MDA-MB-231 tumour growth in vivo ( Supplementary Fig. 21 ). Together, our data indicate that the role of 14-3-3σ in suppressing Myc-promoted glycolysis, glutaminolysis and mitochondrial biogenesis can be recapitulated in vivo . In summary, we discovered that 14-3-3σ opposed and reversed cancer metabolic reprogramming by promoting Myc degradation ( Fig. 9i , Supplementary Fig. 22 ). We also showed that loss of 14-3-3σ was associated with the upregulation of many major cancer hallmarks. Our results additionally elucidated the crosstalk among central cellular processes such as cell cycle, energy metabolism, p53 signalling and Myc network in cancer. Our findings also pointed out that elevating the function of 14-3-3σ in tumours is a potential direction for targeted anticancer metabolism therapies. Metabolic reprogramming has emerged as a new hallmark of cancers. Many oncogenes or tumour-suppressor genes are deregulated, which leads to abnormal cellular bioenergetics that give cancer cells a growth advantage either by providing fuel for cancer cell growth or creating microenvironments that facilitate cancer invasion. Our clinical data, based on PET SUVs, indicate that loss of 14-3-3σ leads to increased glucose uptake in tumours. This finding suggests a functional role for 14-3-3σ in controlling cancer glycolysis. In searching for a potential mechanism behind 14-3-3σ-mediated suppression of the glycolytic pathway, we found Myc to be the main culprit. Our data show that 14-3-3σ is able to downregulate Myc stability by enhancing Myc polyubiquitination. The 14-3-3σ-facilitated destabilization of Myc could regulate cancer energy metabolism through the following mechanisms: (1) by blocking Myc-mediated expression of glycolytic genes; (2) by suppressing Myc-mediated upregulation of genes involved in glutaminolysis and mitochondrial biogenesis. Thus, our results reveal a new regulatory pathway in cancer cell bioenergetics. In addition, 14-3-3σ-Myc axis regulation also provides a new example of the important balance between oncogenes and tumour suppressors in cellular metabolism regulation. 14-3-3σ associated with Myc and promoted Myc interaction with Pin1 (Peptidyl-prolyl cis – trans isomerase NIMA-interacting 1) [39] . Pin1–Myc interaction altered Myc protein structure that allowed Fbxw7 (Myc E3 ubiquitin ligase) to bind to Myc, causing Myc polyubiquitination and subsequent proteosomal degradation [39] , [40] . In our study, we used an inducible system to re-express 14-3-3σ in 14-3-3σ null cell lines. Our data revalidated that 14-3-3σ is a strong regulator for Myc ubiquitination and therefore reduces Myc stability. This 14-3-3σ-mediated downregulation of Myc protein stability translates into effects that negatively affect Myc target gene expression. Some of these genes are involved in glycolysis, glutaminolysis and mitochondrial biogenesis. This important functional link between Myc and 14-3-3σ provides important insight into the relationship between metabolic dysregulation and the frequent loss of 14-3-3σ during tumorigenesis. 14-3-3σ, which has a nuclear exporting signal, binds to c-Myc at the T343 site [39] . It is also possible that 14-3-3σ binds to Myc and facilitates Myc cytoplasmic localization through nuclear exporting signal, which may reduce c-Myc transcriptional activity and enhance c-Myc degradation. This type of regulation has been observed in 14-3-3σ-MDM2, 14-3-3σ-COP1, 14-3-3σ-cyclin B/Cdc2 and 14-3-3σ-cyclin E/CDK4-CDK6 interactions as previously reported in other studies [41] , [42] , [43] , [44] . Our data indicate that the loss of 14-3-3σ leads to elevated lactate production, and that re-expression of 14-3-3σ reduces lactate generation. This elevation of lactate production is caused by upregulation of lactate dehydrogenase A when 14-3-3σ expression is lost. The increase in lactate production due to 14-3-3σ loss enhances the acidification of extracellular environment as shown by our ECAR measurements. Lactate is important for cancer cell invasion and metastasis. It was documented that lactate can significantly enhance cancer cell motility and facilitate the breaking down of extracellular matrix [30] . It has also been shown that lactate stimulates the migration of epithelial cancer cells and can promote cancer metastasis to distant organs. For example, lactate administration fuels lung metastasis in a breast cancer mouse model [31] . Therefore, loss of 14-3-3σ may give cancer cells an advantage in terms of cell migration and metastasis as indicated in our cancer-hallmark characterization. In addition, the fact that 14-3-3σ null cells have a high concentration of ATP means that cancer cells have an edge when it comes to cell growth and drug resistance. This is because ATP is both a major DNA precursor often used for repairing genetic damage and a key energy source for multidrug resistance efflux pumps that discard toxic chemotherapy agents. It has also been reported that glycolytic enzymes play important roles in cancer cell survival. For example, Hexokinase 2 blocks cytochrome c release from mitochondria [45] , [46] , thereby protecting cancer cells from apoptosis. In addition, glucose-6-phosphate isomerase has been shown to stimulate cell motility, an important step in the metastatic process [47] , [48] . Therefore, the fact that loss of 14-3-3σ expression elevates the levels of these glycolytic enzymes could have a tremendous impact not only on tumour bioenergetics but also on other hallmarks of cancers. Myc can drive oxygen consumption, mitochondrial biogenesis and glycolysis. This indicates that Myc stimulates both aerobic glycolysis and mitochondrial oxidative phosphorylation. This phenomenon allows cells with high levels of Myc to adjust to microenvironments with various oxygen levels (both hyper- and hypoxic), freeing them from dependence on oxygen from blood vessels. We have found that loss of 14-3-3σ leads to increased oxygen consumption. More importantly, re-expressing 14-3-3σ can suppress oxygen consumption and mitochondrial biogenesis; this is consistent with the 14-3-3σ-Myc axis regulation. 14-3-3σ expression markedly reduced mitochondrial mass, TFAM level and the expression of mitochondrial genes. This again is the result of 14-3-3σ-Myc axis regulation. This observation is important because mitochondria are not only cellular power stations but also factories that produce many important precursors for amino acid (oxaloacetate, α-ketoglutarate), lipid (citrate), haeme group (succinyl CoA) and nucleotide (oxaloacetate transaminated to aspartate) biosynthesis. Therefore, a strong decline in mitochondrial mass could have a deleterious impact on cancer cell growth. Indeed, our NMR analysis demonstrated that 14-3-3σ expression correlates with a reduction of many key amino acids (for example, methionine, glutamate, glutamine and arginine), phospholipid metabolites and precursors for nucleotide synthesis. It is still unclear whether the reduction in amino acid and phospholipid levels is a direct effect of 14-3-3σ, a consequence of 14-3-3σ-mediated suppression of glycolysis, glutaminolysis and mitochondrial mass, or both. These observations, however, imply that 14-3-3σ has a multifunctional role in cancer cell metabolic control. Furthermore, glutaminolysis is both a major source of metabolites for large-scale biosynthesis and a vital energy source for cancer cells. Myc promotes glutaminolysis by activating the expression of glutamine transporters ( ASCT2 and SN2 ) and glutaminase 1 ( GLS1 ). Glutamine is transported by glutamine transporters and is converted to α-ketoglutarate as a result of an anaplerotic reaction catalysed by glutamate dehydrogenase to replenish biosynthetic intermediates of the TCA cycle. It is important to point out that 14-3-3σ re-expression in 14-3-3σ null cells leads to the reduction of glutamate concentration levels, indicating that 14-3-3σ may also be involved in glutaminolysis. Indeed, our biochemical data show that re-expression of 14-3-3σ in 14-3-3σ null cells can suppress the Myc-activated genes involved in glutaminolysis. Thus, our data indicate that loss of 14-3-3σ leads to Myc activation and widespread derailing of cancer bioenergetics. Importantly, all the roles of 14-3-3σ in limiting glucose uptake, pyruvate–lactate flux, mitochondrial biogenesis and glutaminolysis can be recapitulated in vivo . We used both microPET and MRSI to investigate the role of 14-3-3σ in glycolysis in xenograft tumour models. For the MRSI, we used a hyperpolarized 13 C pyruvate tracer to accurately measure the real-time metabolic flux of pyruvate-to-lactate reaction in xenograft tumour models. This advanced tumour-imaging method is sensitive, safe, noninvasive, nonradioactive and is able to provide deep insight into glycolytic regulation during tumorigenesis [37] , [49] , [50] , [51] . These two independent techniques confirmed the regulatory role of 14-3-3σ in cancer energy metabolism in vivo . In conclusion, our study contributes to further elucidate the complicated regulation of cancer bioenergetics. However, further study is needed to fully elucidate the function of 14-3-3σ. Our mass spectrometry analysis of 14-3-3σ-interacting partners revealed that 14-3-3σ could interact with hundreds of targets. The influences of those interactions on metabolic reprogramming including under the condition of hypoxia are still largely uncharacterized. This could possibly explain the various observations about the impact of 14-3-3σ on tumorigenesis. We believe that more studies are needed to fully understand the complex and multilayered role of 14-3-3σ in normal and cancer cells. In conclusion, our study contributes to further elucidate the complicated control of cancer bioenergetics by identifying 14-3-3σ-Myc as a new regulatory axis of cancer metabolism. Furthermore, these findings suggest that 14-3-3σ could be used as a target in the design of cancer metabolism-targeted therapies [3] . Clinical relevance of 14-3-3σ in breast cancer Breast cancer patients’ tumour and normal breast tissues were stained with anti-14-3-3σ antibodies (1:200 dilution, Fitzgerald Industries International). Immunohistochemical staining results of 14-3-3σ were quantified using a Dako ChromaVision ACIS III system and analysed by the Department of Pathology at the MD Anderson Cancer Center (MDACC). Immunohistochemical staining results of 14-3-3σ in normal breast tissue were used as a reference to classify breast cancer patients into low and normal-high 14-3-3σ groups. There were 60 patients in the low 14-3-3σ group and 25 patients in the normal-high 14-3-3σ group. Overall and relapse-free survival curves were built on the basis of corresponding cancer patients’ clinical records at the MDACC. Immunohistochemical staining Breast cancer tissue microarrays were provided by the Department of Pathology at the MDACC. Xenograft breast tumour slides were constructed by the Histology Core Facility at MD Anderson. Immunohistochemical, haematoxylin and eosin, and cleaved caspase-3 staining were carried out by the Tissue Core Facility at MD Anderson. Other immunohistochemical staining processes were performed according to the protocols provided by the Department of Pathology [29] , [52] , [53] . Tissue microarrays and tumour slides were stained with anti-14-3-3σ (1:200 dilution) and anti-c-Myc (1:50 dilution). Immunohistochemical staining results were analysed by pathologists of the Department of Pathology and quantified by using a Dako ChromaVision System ACIS III in the Department of Molecular and Cellular Oncology. Immunohistochemical staining score (arbitrary unit, a.u.) is the product of immunhistochemical staining intensity multiplied by percentage of the brown area. The IHC expression score is defined by this formula: IHC expression score=intensity of IHC staining (within the tumour area) × area of IHC staining (within the tumour area). The intensity and area of IHC staining were calculated using the Dako ACIS III Imaging Station slide scanner. The whole-tumour tissue microarrays were scanned using this slide scanner. Tumour locations were determined on the basis of pathological observations. The intensity and area of IHC staining within tumour areas were calculated using the Dako ACIS III Imaging Station software. Bioinformatics analysis Breast cancer patient data sets GSE20194, GSE5847, GSE2109, GSE11121, among others were downloaded from the Oncomine, The Cancer Genome Atlas and Gene Expression Omnibus databases. These cohorts were analysed by Gene Set Enrichment Analysis (Broad Institute), Nexus Expression 3 (BioDiscovery), Gene Spring 12 (Agilent Technologies) and Ingenuity Pathway Analysis (Ingenuity Systems). A Circos map of the data (Circos Software, Circos.ca) analysis [54] revealed that downregulation of 14-3-3 was associated with an increase in cancer hallmarks and their related biological processes. The GSE20194 cohort, which includes 255 patients with stage I–III breast cancer who had not received any treatment at the time of sample collection, was chosen for tumour analysis. Breast tumour biopsies from this cohort were collected by fine-needle aspiration, with minimal contamination by normal tissues. 14-3-3σ expression in the tumours was quantified using the microarray analysis. 14-3-3σ expression of normal breast tissues was used as a reference to select the tumours that were in the highest (high) or lowest (low) 14-3-3σ quartile. The cohort included 64 patients with high 14-3-3σ and 63 with low 14-3-3σ. Tissue culture Breast cancer cell lines MDA-MB-231, MDA-MB-435 and T47D; normal breast epithelial cell line MCF10A; and lung cancer cell line H1299 were purchased from American Type Tissue Collection and were grown in high-glucose DMEM supplemented with 10% fetal bovine serum (FBS; Sigma-Aldrich, Atlanta Biologicals, Georgia, USA), 2 mM L-glutamine (Cellgro) and 1% antibiotic–antimycotic solution (Invitrogen). Colon cancer cells HCT116 14-3-3σ +/+ (wild type (WT)), 14-3-3σ −/− and p53 −/− (a kind gift from Dr Bert Vogelstein’s research group) were cultured in the same high-glucose DMEM containing the same supplements. All cells were grown in an incubator at 37 °C in a humidified atmosphere containing 5% CO 2 . MDA-MB-231 and HCT116 WT, HCT116 14-3-3σ −/− and HCT116 p53 −/− cell lines carrying a tet-On Flag-14-3-3σ system were cultured in high-glucose DMEM containing 10% tetracycline-free FBS (Atlanta Biologicals), 2 mM L-glutamine and 1% antibiotic–antimycotic solution. Metabolomics analysis using NMR HCT116 14-3-3σ +/+ , HCT116 14-3-3σ −/− , HCT116 14-3-3σ −/− infected with Ad-βgal and HCT116 14-3-3σ −/− infected with Ad-14-3-3σ were grown under culture conditions [26] , [55] for 48 h. A sample of cells (20 × 10 6 ) from each cell line was collected and snap-frozen with liquid nitrogen. Total metabolites were then extracted from cell pellets using freeze–thaw extraction and filtration protocols provided by Chenomx Inc. Metabolite extracts were snap-frozen with liquid nitrogen and shipped to Chenomx Inc. on dry ice for NMR analysis. Data were analysed using the Chenomx NMR software and are displayed as heat maps generated by the Cluster and Java Treeview programmes. Cell pellet collection procedure : For each plate, 20 million cells were rapidly collected by trypsinization and were centrifuged at 280 g for 5 min at 4 °C. Each cell pellet was washed with 40 ml of ice-cold PBS, followed by centrifugation at 280 g for 5 min at 4 °C. PBS was removed by vacuum. Each cell pellet was resuspended in 1 ml of ice-cold PBS and transferred to a 1.5-ml conical tube. Centrifugation was carried out at 1,700 g (maximal speed without causing damage to cellular structures) for 5 min at 4 °C. PBS was removed by vacuum using fine tips. All cell pellets were then snap-frozen using liquid nitrogen and stored at −80 °C until metabolite extraction steps. Cell lysis procedure using the freeze–thaw method : Cell pellets were removed from −80 °C freezer and thawed on ice. Thawed cell pellets were resuspended in 500 μl of 500 μM phosphate buffer (pH 7.0). Cell samples were then snap-frozen in liquid nitrogen and then slowly thawed on ice. Cell samples were sonicated for 30 s on ice. Cell samples were snap-frozen in liquid nitrogen and then slowly thawed on ice. Cell samples were centrifuged at 13,793 g for 10 min at 4 °C. Cell lysates (10 μl) were used for protein concentration measurement (for normalization purpose). Metabolite extraction procedure : Cell samples were filtered through a prewashed Nanosep 3 K Omega microcentrifuge filter tube (Pall Corporation, Catalog # OD003C33) by centrifuging for 15–30 min at 13,793 g at 4 °C for 30 min or until the maximum amount of sample was accumulated. Filtered samples were transferred to new vials and labelled, and snap-frozen by liquid nitrogen. Samples were shipped to the analysis site on dry ice. NMR data were analysed using Chenomx NMR Suite ( www.chenomx.com ). Heat map was built using the Cluster and Treeview software. Establishment of retroviral tet-On 14-3-3σ systems Flag-14-3-3σ cDNA was amplified using PCR from a pCMV5-Flag-14-3-3σ plasmid in Dr Lee’s laboratory and cloned into a pRetro-CMV/TO retroviral plasmid (kindly provided by Dr L.M. Staudt, National Cancer Institute). After sequence verification, the pRetro/CMV-TO-Flag-14-3-3σ plasmid was co-transfected with VSVg and Gag/Pol plasmids into 293T cells to produce 14-3-3σ tet-On retroviruses. Tet repressor retroviruses were produced from the 293T cells after co-transfection of p-BMN-TetR-BSR, VSVg and Gag/Pol plasmids (also provided by Dr Staudt). Cells of interest were first infected with TetR-BSR retroviruses and then selected with appropriate culture medium containing 20 μg ml −1 blasticidin for 1 week. Selected cells were infected with retroviruses carrying Flag-14-3-3σ and were subjected to a second selection with 5 μg ml −1 puromycin for 1 week. The culture media for cells with the retroviral tet-On system are DMEM High glucose (Hyclone Laboratories, Utah, USA; Catalogue #SH30243.01) and I-1640 (Hyclone Laboratories; Catalog #SH30027.01) supplemented with 2 mM L-glutamine, and 1% antibiotic–antimycotic solution. The FBS for growing cells carrying tet-On system is tetracycline-free (tetracycline-tested) FBS from Atlanta Biologicals (Catalogue #S10350). All culture media for maintaining cancer cells infected with tet-On Flag-14-3-3σ retroviruses contain 10 μg ml −1 Blasticidine (Invivogen, CA, USA; Catalogue #ant-bl-1) to ensure the continuous expression of the fusion protein Tet repressor—Blasticidine-resistant protein, which is important for the tight control of Flag-14-3-3σ expression, and 2 μg ml −1 Puromycin (Invivogen; Catalogue #ant-pr-1) to keep Flag-14-3-3σ gene presence. For in vivo studies, MDA-MB-231 tet-On 14-3-3σ breast cancer cells were injected into the mammary fat pad of female nude mice. Tumour growth was monitored for 4 weeks. Tumour-bearing mice were divided into two groups of 5–10 mice, an experimental and a control group. To induce 14-3-3σ expression in vitro , doxycycline (a stable derivative of tetracycline) [56] was added to the culture medium at a final concentration of 5 ng ml −1 for 48, 72 or 96 h. The culture medium with doxycycline was replaced daily to induce Flag-14-3-3σ expression. To induce 14-3-3σ expression in xenografts in vivo , mice in the experimental group were given doxycycline in their drinking water (final concentration 200 μg ml −1 ) for 2 weeks. Because of the sensitivity to light and short half-life of doxycycline, the drinking water with doxycycline was contained in opaque bottles and replaced with a freshly prepared solution every 48 h. The control group received plain drinking water without doxycycline. Lentiviral shRNA knockdown of 14-3-3σ and c-Myc 14-3-3σ and c-Myc shRNA lentiviral plasmids were purchased from Sigma-Aldrich. 14-3-3σ and c-Myc shRNA lentiviruses were then produced from 293T cells following a protocol similar to that used for the tet-On Flag-14-3-3σ system. Infection efficiency was enhanced by adding 8 μg ml −1 Polybrene and subjecting the cells to centrifugation at 2,000 r.p.m. for 60 min at 32 °C. Knockdown efficiency was verified using western blot analysis. Extracellular acidification and OCR Cancer cell lines containing the retroviral 14-3-3σ tet-On system were maintained in the growth medium already described. The other cancer cell lines were maintained in a different growth medium: high-glucose DMEM containing 10% normal FBS, 2 mM L-glutamine and 1% antibiotic–antimycotic solution. Oligomycin, an inhibitor of ATP synthase, was prepared from 1,000 × stock at a concentration of 10 mM in dimethyl sulfoxide (DMSO). FCCP, an ionophore and strong mitochondrial depolarizer, was prepared from 1,000 × stock at a concentration of 5 mM in DMSO. Rotenone, a potent inhibitor of mitochondrial complex I, and antimycin A, a strong suppressor of mitochondrial complex III, were solubilized from 1,000 × stock solutions at concentrations of 10 mM in DMSO. To measure ECAR and OCR, 3 × 10 4 cells from each cell line were seeded into each well of a XF24 microplate 16 h before the experiment. Right before the assays, these cells were changed from a culture medium to an assay medium (low-buffered DMEM containing 25 mM D-glucose, 1 mM sodium pyruvate and 1 mM L-glutamine) and incubated for 1 h at 37 °C. OCR and ECAR were measured using a Seahorse Extracellular Flux Analyser (Seahorse Biosciences). After baseline measurements, 75 μl of the above-mentioned inhibitors prepared in the assay medium were sequentially injected into each well to reach the final working 1 × concentrations. After 5 min of mixing to equally expose cancer cells to the chemical inhibitors, OCR and ECAR were measured again. Data were analysed using the Seahorse XF software. OCR is reported in pmole min −1 , ECAR in mpH min −1 . OCR and ECAR measurements were normalized to either final cell number or protein concentration. Lactate production and glucose consumption assays In these assays, HCT116 WT, HCT116 14-3-3σ −/− , HCT116 Luciferase shRNA, HCT116 14-3-3σ shRNA #419, HCT116 14-3-3σ shRNA #483, HCT116 14-3-3σ −/− TetR 14-3-3σ and MDA-MB-231 TetR 14-3-3σ cells were plated with the same number (200,000 cells per well in six-well plates). After 48 h, the medium was collected for measuring lactate and glucose concentrations. Lactate concentrations were measured with an Accutrend Lactate Analyzer (Roche Diagnostics). Glucose consumption was determined by measuring the difference in glucose concentrations at the beginning and the end of experiments. The glucose level was quantified by using a Freestyle Glucose Meter (Abbott Laboratories). The final live cell numbers were counted using hemocytometer and Trypan Blue staining. Lactate production and glucose consumption were normalized to the final number of live cell and culture time. Glucose uptake in cells was quantified by using (2-( N -(7-nitrobenz-2-oxa-1,3-diazol-4-yl)amino)-2-deoxyglucose (2-NBDG)), a green fluorescent glucose analogue (Molecular Probes, Invitrogen). Experimental cells were incubated in glucose-free DMEM with 10% FBS containing 120 μM 2-NBDG for time intervals ranging from 0 to 3 h. 2-NBDG uptake was analysed by using a fluorescent microscope (Olympus) and a FACS Canto flow cytometer (BD Biosciences). Flow cytometry data were analysed using a FlowJo X software (FlowJo). ATP production ATP concentration was measured using the ATP Bioluminescence Kit CLS II (Roche) following the manufacturer’s protocol. The principle of ATP Bioluminescence Kit relies on the following luciferase-catalysed reaction: ATP+D-luciferin+O 2 →oxyluciferin+PPi+AMP+CO 2 +light. The bioluminescent signal from this reaction is proportional to the ATP concentration and measured by a Clarity Luminescence Microplate Reader (BioTek). A standard curve with known ATP concentrations was used to determine the actual ATP levels in samples. Glutaminolysis assay Glutaminolytic activity in cells was measured by using a glutaminolysis assay kit (Sigma-Aldrich, Catalogue #AA0100-1KT) that measures ammonia production as a surrogate for glutaminolysis. In this assay, L-glutamate dehydrogenase specifically catalyses the reaction to convert ammonia and α-ketoglutaric acid to form L-glutamate. This biochemical reaction rapidly reduces NADPH, and also oxidizes NADP + . The oxidation of NADPH, which is correlated and associated with the ammonia concentrations, leads to a reduction in absorbance at 340 nm. This decrease in absorbance at 340 nm is detected and quantified using spectrophotometers. Mitochondrial mass measurement assays Mitochondrial mass was quantified by staining with MitoTracker Green FM (Molecular Probes, Invitrogen) and was analysis with a FACS Canto flow cytometer (BD Biosciences). MitoTracker Green FM is a green fluorescent dye associated with functional mitochondria. Flow cytometry data were analysed using a FlowJo X software (FlowJo). Western blot analysis Cells and tumour samples were subjected to lysis using a standard lysis buffer containing NP-40 and 0.1% Triton X-100. The antibodies used in this study included anti-Flag (Sigma-Aldrich, clone M2, catalogue #F1804-1MG), anti-actin (Sigma-Aldrich, catalogue #A2066), anti-hexokinase 2 (Cell Signaling Technology, catalogue #2867), anti-aldolase (Cell Signaling Technology, catalogue #3188), anti-pyruvate kinase M2 (Cell Signaling Technology, catalogue #3198), anti-lactate dehydrogenase A (Cell Signaling Technology, catalogue #3582; Epitomics, catalogue #3468-1), anti-pyruvate dehydrogenase kinase 1 (Zymed, catalogue #34-9,500), anti-enolase 1 (Cell Signaling Technology, catalogue #3810), anti-glutaminase (Abcam, catalogue #ab60709), anti-phosphofructose kinase 1 (Novus Biologicals, catalogue #NBP1-19585), anti-phosphoglucose mutase 1 (Abcam, catalogue #ab55616), anti-14-3-3σ (Fitzgerald Industries International, catalogue #10R-S101a) and anti-c-Myc (Abcam, clone 9E10, catalogue #ab32). Original films of immunoblotting were in supplementary Figs 24–29 . Real-time PCR For quantitative real-time PCR, total RNA was collected by using Trizol Reagent (Invitrogen), and cDNA was synthesized by using an iScript cDNA Synthesis Kit (Bio-Rad). Real-time PCR was performed using iQ-SYBR Green Supermix (Bio-Rad), StepOnePlus Real-time PCR platform (Applied Biosystems Inc.) and iCycler CFX96 Real-time PCR Detection System (Bio-Rad). Actin and 18S rRNA were used as internal references for normalization. The nucleotide sequences of the primers used for real-time PCR were listed in Supplementary Table 4 . Ubiquitination assay Human HCT116 14-3-3σ −/− , MDA-MB-231, HCT116 p53 −/− and H1299 cells carrying retroviral a tet-On Flag-14-3-3σ system were used for the assay. MG132 (10 mM; Sigma-Aldrich, St Louis, MO, USA, Catalogue #M7449) was added to the culture media for 8 h for blocking proteasome-mediated protein degradation [57] , [58] to facilitate the accumulation of ubiquitinated proteins. NP-40-containing lysis buffer was used for cell lysis. N -Ethylmaleimide (5 mM; Sigma-Aldrich, Catalogue #E3876) was added to NP-40-containing lysis buffer to inhibit deubiquitinases and prevent deubiquitination. The ubiquitinated c-Myc protein was immunoprecipitated with monoclonal anti-c-Myc antibody (Sigma-Aldrich, 9E10 clone, Catalogue #M4439) and subsequently immunoblotted with monoclonal mouse antiubiquitin antibody (Life Technologies, USA, Catalogue #13-1,600). Dual-luciferase reporter assay c-Myc transactivational activity was measured by using a Dual-Luciferase Reporter Assay System (Promega) with a luciferase reporter plasmid containing a TERT (telomerase reverse transcriptase) promoter. TERT is a c-Myc target gene and its promoter contains an E-box c-Myc-binding site. microPET scan Seven-week-old female nude mice bearing MDA-MB-231 tet-On 14-3-3σ breast cancer xenografts were imaged with a MicroPET Rodent–R4 scanner for 30 min after injection with 400 μCi 18 FDG according to an imaging protocol used by the Small Animal Imaging Facility of MD Anderson. Tumours were also visualized with a Burker 7.0 Tesla magnetic resonance imager according to the facility’s standard imaging procedures. The details of microPET Scan were described as below: the MicroPET R4 system was used for these mouse imaging studies. The PET images were acquired with energy windows set at 350–650 keV (for better scatter rejection). Coincidence timing window was set at 6 ns. Animals were sequentially scanned. Each animal was injected ∼ 0.4 μCi 18 FDG radiotracers, with around 2.7 μCi cm −3 concentration. It was followed by a 30-min uptake time while the animal was put in cage with little movement to reduce the muscle update. Each image was acquired 30 min per bed position. Image data were analysed with the ASIPro VM mciroPET imaging analysis software. The image-quantitation calibration was measured with a uniform phantom with known activity concentration. A representative chart of imaging workflow is included ( Supplementary Fig. 23 ). Three different ratios were calculated on the basis of the maximal, minimal and mean values of image intensities measured within the selected region of interest. In this imaging experiment, when we compared the images of the control mice (without Flag-14-3-3σ induction) with those of the treated mice (with Flag-14-3-3σ induction), there was a consistent 2:1 reduction in lesion/background image intensity ratios. The mean-calculated lesion (tumour)/background (normal tissue) ratios, which are more representative with less bias of single pixel value domination, were used to build our graphs. 13 C hyperpolarization A mixture containing 20 μl (26 mg) of [ 13 C]pyruvic acid (Cambridge Isotopes) with 15 mM of trityl radical OX063 (GE Healthcare) was combined with 0.6 μl 50 mM Prohance (Bracco Diagnostic Inc.) and polarized using a Hypersense DNP system (Oxford Instruments). In brief, the solution was frozen to ∼ 1.4°K and irradiated at 94.154 GHz for 45–60 min in a 3.35-T magnetic field. When the solid-state polarization reached a plateau, the solution was dissolved in 4 ml of a heated (180 °C) solution containing 80 mM NaOH and 50 mM NaCl. The final solution containing 80 mM hyperpolarized pyruvate at a nominal temperature of 37 °C and pH of 7.6 was flushed into a receptacle from which 200 μl was drawn for injection. The injection was administered to tumour-bearing and control mice over 10 s beginning within 12 s of sample dissolution. Magnetic resonance spectroscopy Animals were anaesthetized using 0.5–5% isoflurane in oxygen and then placed on a positioning sled with built-in channels for distribution of anaesthesia gases and circulation of warm water to maintain animal temperature. The chemical fate of the hyperpolarized [ 13 C]-pyruvate was monitored using a 7T Biospec USR7030 system (Bruker Biospin MRI Inc.) with a dual-tuned 1 H– 13 C volume coil with 72-mm inner diameter and a custom-built 13 C surface coil (12 mm inner diameter) placed over the tumour. Animal position was confirmed by using a three-plane gradient-echo proton MRI sequence (TE=3.6 ms, TR=100 ms, 30° excitation angle), and the location of the tumour was confirmed in T2-weighted axial and coronal spin-echo images (TE=50 ms, TR=2,500 ms, 1-mm slice thickness, 4 cm × 3 cm field-of-view encoded over a 256 × 192 matrix in 1-mm sections). Field homogeneity was maximized over the tumour volume using a point-resolved spectroscopy sequence. For 13 C measurements, a signal was generated by the volume coil and detected using the surface coil. Dynamic spectra were acquired by using a slice-selective single-pulse sequence (SW=5,000 Hz over 2,048 points, 10° excitation, 8-mm slice thickness) that was repeated every 2 s for 3 min beginning just before injection of 13 C via tail-vein catheter. The spectra were phase-adjusted, and the area under the spectral peaks corresponding to the C1 of pyruvate and lactate were integrated to generate curves describing the arrival of hyperpolarized pyruvate and its conversion into hyperpolarized lactate. These curves were fit to kinetic models that account for chemical conversion. The model we used is a modification from the one described in ref. 38 . Our model has two physical compartments to separate the effects of tracer circulation, extravasation and activity. All modelling was performed by using Matlab (The Mathworks). Statistical analyses All bar graphs and line graphs represent means±95% confidence intervals or s.d.’s unless otherwise stated. The error bars of ECAR and OCR line graphs from Seahorse Extracellular Flux Analyser are s.d.’s. Student’s t -test was used to compare differences between two groups. One-way analysis of variance was employed for comparison if there were more than two groups, unless otherwise stated. A P value less than 0.05 was considered to represent a statistically significant difference. Pearson correlation was used to identify positive and negative correlations between 14-3-3σ expression and expression of other genes. The log-rank (Mantel–Cox) test was used to compare survival times of breast cancer patients. Data were analysed using Prism (GraphPad software) and Sigma Graph (Systat Software) unless otherwise noted. All experiments were independently repeated at least four times. Compliance information All experiments involving cancer patient samples and information were conducted under clinical protocols approved by the Institutional Review Board of The University of Texas MDACC. All experiments and procedures involving animals were approved by the Institutional Animal Care and Use Committee of MD Anderson, which is accredited by the Association for the Assessment and Accreditation of Laboratory Animal Care International. How to cite this article: Phan, L. et al . The cell cycle regulator 14-3-3σ opposes and reverses cancer metabolic reprogramming. Nat. Commun. 6:7530 doi: 10.1038/ncomms8530 (2015).